Contact-induced clustering of syntaxin and munc18 docks secretory granules at the exocytosis site Docking of secretory vesicles at the plasma membrane is a poorly understood prerequisite for exocytosis. Current models propose raft-like clusters containing syntaxin as docking receptor, but direct evidence for this is lacking. Here we provide quantitative measurements of several exocytosis proteins (syntaxin, SNAP25, munc18, munc13 and rab3) at the insulin granule release site and show that docking coincides with rapid de novo formation of syntaxin1/munc18 clusters at the nascent docking site. Formation of such clusters prevents undocking and is not observed during failed docking attempts. Overexpression of syntaxins’ N-terminal Habc-domain competitively interferes with both cluster formation and successful docking. SNAP25 and munc13 are recruited to the docking site more than a minute later, consistent with munc13’s reported role in granule priming rather than docking. We conclude that secretory vesicles dock by inducing syntaxin1/munc18 clustering in the target membrane, and find no evidence for preformed docking receptors. Exocytosis is a fundamental cellular process that fuses intracellular vesicles with the plasma membrane and is involved in secretion, protein trafficking and membrane repair. Exocytosis of neurotransmitter- and hormone-containing secretory vesicles is triggered within milliseconds by a rise in cytosolic Ca 2+ . To achieve this temporal precision, a pool of release-ready vesicles is morphologically docked at the plasma membrane with the exocytosis machinery in place [1] , [2] , [3] , [4] , [5] , [6] . Sustained secretion therefore requires tethering and docking of new vesicles at the plasma membrane followed by a set of slower priming reactions that render docked vesicles fusion-competent [1] , [3] . In most secretory cells only a small fraction of secretory vesicles or granules is in the release-ready state. For example, a typical pancreatic β-cell stores at least a day’s worth of insulin, but only 1% of its granules undergo exocytosis immediately upon stimulation [7] , [8] . Systemically, this underlies the biphasic nature of insulin secretion, which is important for insulin action [9] . In neuroendocrine cells, docked secretory vesicles are stationary at the plasma membrane [2] , [10] , [11] , consistent with their physical binding to specialized docking structures. The molecular steps leading to the docked state are not well understood, but several core exocytosis proteins appear to be required for docking in addition to their role in the membrane fusion step. These include the soluble N-ethylmaleimide-sensitive factor attachment protein receptor (SNARE) syntaxin 1 (refs 12 , 13 , 14 ) and its binding partner, the Sec1/Munc18 protein munc18 (refs 15 , 16 , 17 , 18 ). In addition there is evidence for involvement of the cognate SNAREs synaptobrevin [19] and SNAP25 (refs 16 , 19 ), the Ca 2+ sensor of exocytosis synaptotagmin [16] , [20] , and rab GTPases and their effectors [21] , [22] , [23] . The latter can indirectly bind syntaxin via munc18, and such complexes have been proposed to target secretory granules to the plasma membrane [22] . Other possible interactions between granule and plasma membrane involve binding of the vesicle SNARE synaptobrevin to binary syntaxin/SNAP25 complexes [24] and binding of synaptotagmin to acidic phospholipids such as phosphatidylinositol 4,5-bisphosphate (PIP2) and phosphatidylinositol 3,4,5-trisphosphate (PIP3) [25] , [26] , [27] . At the docking site, SNARE proteins aggregate in 50–60 nm wide raft-like clusters that contain 50–70 syntaxin and a similar number of SNAP25 molecules [28] , [29] , [30] , [31] , [32] . These sites are enriched in PIP2 and PIP3, which affect clustering of syntaxin 1A through interaction with positively charged residues near its transmembrane domain [27] , [33] , [34] . Since there are multiple possible interactions between syntaxin and the granule, syntaxin-containing clusters in the plasma membrane have been proposed as docking receptor for the incoming vesicle [16] , [19] , [26] , [35] . Here we image protein recruitment to the docking site to test a crucial requirement of this model, namely that syntaxin clusters must exist at the docking site before arrival of the vesicle. We provide the first quantitative time course of protein recruitment to the docking site and show that rapid recruitment of syntaxin1 and munc18 to the contact site converts secretory vesicles from loosely tethered to the stably docked state, which is required for exocytosis. Loosely tethered and stably docked granules We imaged docking of insulin-containing secretory granules by high-resolution total-internal reflection microscopy (TIRF-M) [36] . Individual docking events were readily observed in cells expressing the granule marker neuropeptide-Y (NPY)-mCherry ( Fig. 1a ). When a granule approached the plasma membrane, its fluorescence increased as it reached the TIRF-illuminated volume. Many granules arrived and then became arrested after reaching their highest brightness, likely because they became bound to the plasma membrane. However, not all granules remained immobilized at the plasma membrane. Residence times were bimodally distributed ( Fig. 1b ), and about two-thirds of the arriving granules returned to the cytosol within 25 s ( Fig. 1c ). This suggests the presence of a loosely tethered state that allows granules to undock at a rate of 0.12 s −1 . In the following we refer to the two groups of granules as ‘stably docked’ (>25 s) and ‘visitors’ (<25 s). Particle tracking analysis confirmed this conclusion; granules with short residence times (<25 s) retained higher mobility at the docking site, measured as caging diameter, than those with long residence times >25 s ( Fig. 1d,e ). Since visiting events were rare and their duration short (8.6 s and 0.08 μm −2 min −1 , Fig. 1b ), we estimate that at any time only ~2% of all the granules visible by TIRF (density 0.6 μm −2 ) represent visitors. About 6% of the visible granules docked stably during the previous minute. 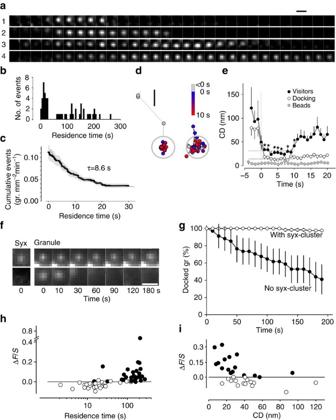Figure 1: Stable docking requires clustered syntaxin. (a) Image sequences showing four secretory granules (gr) labelled with NPY-cherry during their approach to the plasma membrane, frames are 1 s apart. Granules 1–3 remain <20 s at the membrane, while granule 4 remained in place throughout the experiment. Scale bar, 1 μm. (b) Histogram of the granule residence times at the plasma membrane for all incoming granules as in A (83 granules; shown as average and s.e.m. of 9 cells). (c) Scaled survival plot of data ina,b, normalized for cell area and observation time. The overlay is a monoexponential function with a decay constant of 8.6 s. (d) Trajectories of two granules during their first 10 s at the plasma membrane. Residence times were 18 (left) and >73 s (right). The circle is centred on the average granule position during 0–10 s. Scale bar, 100 nm. (e) Quantification of caging diameter (CD, defined as average distance of the granule from its average position 0–10 s after arrival) of granules at the plasma membrane, for visitors (residence times 10–20 s, black) and stable docking events (residence times >25 s, hollow); 17 granules each in 7 cell. Immobilized fluorescent beads (100 nm diameter, similar brightness as granules) were recorded with identical camera settings (grey); average CD was 7±2 nm (n=10). Note that stably docking granules became immobilized while visitors retain higher mobility throughout. (f) Two examples of granules (gr) and associated syntaxin-EGFP (syx) at various timepoints as indicated; each square is 1.1 μm wide. The upper granule carried a syntaxin cluster and remained docked, while the lower lacked syntaxin and undocked after 10 s. Scale bar, 1 μm. (g) Survival function of docked granules as inf, for 127 granules with syntaxin cluster (hollow) and 95 without (solid); 8 cells. Granules were selected and syntaxin clusters scored in the first frame. All points ≥50 s were significantly different in the two groups (P<0.05). (h) Quantification of syntaxin at the docking site (ΔF/S), as function of granule residence time. Spearman correlation coefficientrs=0.76,P=3 × 10−12. (i) Plot of ΔF/Sfor syntaxin as function of granule CD. Same granules as inh, except for those that could not be reliably tracked due to the close vicinity of neighbouring granules.rs=−0.43,P=3 × 10−4. Inh,ithe average ΔF/Svalues during the first 5 s after granule arrival are shown, for 7 cells. Black circles indicate granules that colocalized with a syntaxin cluster, hollow circles those that did not. Figure 1: Stable docking requires clustered syntaxin. ( a ) Image sequences showing four secretory granules (gr) labelled with NPY-cherry during their approach to the plasma membrane, frames are 1 s apart. Granules 1–3 remain <20 s at the membrane, while granule 4 remained in place throughout the experiment. Scale bar, 1 μm. ( b ) Histogram of the granule residence times at the plasma membrane for all incoming granules as in A (83 granules; shown as average and s.e.m. of 9 cells). ( c ) Scaled survival plot of data in a , b , normalized for cell area and observation time. The overlay is a monoexponential function with a decay constant of 8.6 s. ( d ) Trajectories of two granules during their first 10 s at the plasma membrane. Residence times were 18 (left) and >73 s (right). The circle is centred on the average granule position during 0–10 s. Scale bar, 100 nm. ( e ) Quantification of caging diameter (CD, defined as average distance of the granule from its average position 0–10 s after arrival) of granules at the plasma membrane, for visitors (residence times 10–20 s, black) and stable docking events (residence times >25 s, hollow); 17 granules each in 7 cell. Immobilized fluorescent beads (100 nm diameter, similar brightness as granules) were recorded with identical camera settings (grey); average CD was 7±2 nm ( n =10). Note that stably docking granules became immobilized while visitors retain higher mobility throughout. ( f ) Two examples of granules (gr) and associated syntaxin-EGFP (syx) at various timepoints as indicated; each square is 1.1 μm wide. The upper granule carried a syntaxin cluster and remained docked, while the lower lacked syntaxin and undocked after 10 s. Scale bar, 1 μm. ( g ) Survival function of docked granules as in f , for 127 granules with syntaxin cluster (hollow) and 95 without (solid); 8 cells. Granules were selected and syntaxin clusters scored in the first frame. All points ≥50 s were significantly different in the two groups ( P <0.05). ( h ) Quantification of syntaxin at the docking site (Δ F/S ), as function of granule residence time. Spearman correlation coefficient r s =0.76, P =3 × 10 −12 . ( i ) Plot of Δ F / S for syntaxin as function of granule CD. Same granules as in h , except for those that could not be reliably tracked due to the close vicinity of neighbouring granules. r s =−0.43, P =3 × 10 −4 . In h , i the average Δ F/S values during the first 5 s after granule arrival are shown, for 7 cells. Black circles indicate granules that colocalized with a syntaxin cluster, hollow circles those that did not. Full size image The stably docked state requires clustered syntaxin As in previous work [30] , [31] , [33] , [36] , the majority of docked granules colocalized visually with diffraction-limited clusters of co-expressed syntaxin 1A (syx)-enhanced green fluorescent protein (EGFP), which appeared superimposed onto a hazy background of syx-EGFP fluorescence (see Supplementary Fig. 1A,D–F) . Few of the syntaxin clusters were not colocalized with a fluorescent granule, perhaps reflecting that most but not all granules were labelled ( Supplementary Fig. 1A,E ). In movies (0.1 Hz) of granules and syx-EGFP, association with a syntaxin cluster essentially prevented undocking ( Fig. 1f,g ), suggesting that the clusters stabilize the docked state. Binding of syx-EGFP to the docking site was also quantified using image analysis [36] . The goal was to separate granule-related fluorescence (on-granule, ‘bound’) from unrelated fluorescence in the surrounding area (off-granule, ‘free’). We quantified on-granule fluorescence in a circle ( c ) centred on the granule and subtracted the fluorescence from a surrounding annulus ( a ); the result Δ F=c−a estimates the fluorescence originating from granule-associated syx-EGFP. Positive Δ F values indicate that syntaxin is concentrated at the granule, while negative values indicate exclusion. Off-granule fluorescence was obtained by subtracting out-of-cell-background ( bg ) from a ; the result S=a−bg is proportional to the concentration of free syntaxin molecules unaffected by any granule. See Supplementary Fig. 1H for illustration and Methods for details. Much like in binding assays of classical biochemistry, the relationship of on- and off-granule fluorescence follows a simple one-site binding model [30] in the form The initial slope (Δ F/S for S ≪ K d ) is proportional to the binding affinity ( B max /K d ) of syntaxin to the granule site; see ref. 36 and Supplementary Fig. 1G . Consistent with a role of syntaxin clusters in stabilizing the docked state, Δ F/S for individual granules was positively correlated with the residence time at the plasma membrane ( Fig. 1h ), and negatively correlated with the caging diameter ( Fig. 1i ). The data were also analysed by letting a blinded observer decide whether a cluster was present or not (black and hollow circles in Fig. 1h,i , respectively), confirming the correlations observed using the Δ F/S parameter. Thus, association with a syntaxin cluster distinguishes stably docked granules from those that are loosely tethered. Exocytosis occurs from stably docked granules Traditionally, secretory granules are thought to dock before becoming release-ready [1] , [2] , [3] , but this has been questioned by reports of granule fusion immediately after arrival at the plasma membrane (crash fusion) [12] . We therefore tested whether stable docking was required for stimulated exocytosis in our cells. NPY-EGFP was used as granule marker, which resulted in a characteristic fluorescent transient during exocytosis due to pH-dependent unquenching of the EGFP label [2] . Cells were imaged for >30 s before stimulating exocytosis by exposing to elevated K + , leading to depolarization and Ca 2+ influx. All of the 68 granules undergoing exocytosis were present already in the starting frame of the experiment, and consequently the fluorescence at the release site was constant before exocytosis ( Fig. 2a–c ). No visitor granule exocytosed. In contrast, at least 19 of the remaining granules showed movement, but none of these underwent exocytosis ( Supplementary Fig. 2A ). In Ins1 and many other cells, only a fraction of the docked granules is release-ready and can undergo exocytosis immediately after stimulation [2] , [4] . These granules are often referred to as primed or readily releasable pool (RRP). Indeed, only 6% of the docked granules exocytosed during the single stimulus, although the RRP was emptied ( Supplementary Fig. 2B ). In agreement with previous work [1] , [2] , [3] , [4] we conclude that only stably docked granules exocytose under these conditions, and that the RRP is a small subset of the docked granules. 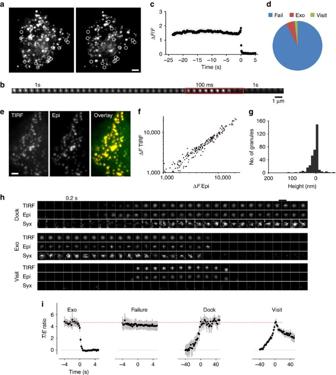Figure 2: Exocytosis occurs only from docked granules. (a) NPY-EGFP expressing cell before (left) and after (right) stimulation with 75 mM K+. Scale bar, 2 μm. Circles indicate positions of granules that exocytosed. Scale bar, 2 μm. (b) Image sequence showing a single granule undergoing exocytosis; 1 or 0.1 s between images, as indicated. (c) Quantification of experiments ina,b. Average fluorescence time course of all exocytosis events (ΔF), aligned to the time of exocytosis and normalized to cell brightness (F); 68 granules in 8 cells. (d) Quantification of docking, visiting, exocytosis and failures ina,b. (e) NPY-cherry-expressing cells imaged in TIRF and Epi mode, and colour overlay as indicated. The TIRF image was acquired 50 ms after the Epi image. Scale bar, 2 μm. (f) Scatterplot of the TIRF versus Epi signals at granules (ΔF). Each point represents a granule. (g) Histogram of the TIRF/Epi ratio for the data inf, scaled as height from the coverslip using a decay constant of 100 nm and assuming that the peak represents granules touching the plasma membrane. (h) Cells expressing NPY-cherry (TIRF, Epi) and syntaxin-EGFP (Syx) were imaged in TIRF and Epi mode and stimulated with K+. Examples of docking, exocytosis (exo) and visiting events are shown. The syntaxin signal was acquired 100 ms before the granule images. Scale bar, 1 μm. To emphasize changes in granule-associated fluorescence, the image sequences were linearly scaled for best contrast. (i) Quantification of the TIRF/Epi ratio for granules as inh. The TIRF ΔFsignal was divided by the average Epi ΔFsignal during 5 s before (exocytosis, failures) or after (docking, visiting) the event. Failures are time-matched granules that did not undergo exocytosis. Data from 20–49 granules in 5–11 cells. Figure 2: Exocytosis occurs only from docked granules. ( a ) NPY-EGFP expressing cell before (left) and after (right) stimulation with 75 mM K + . Scale bar, 2 μm. Circles indicate positions of granules that exocytosed. Scale bar, 2 μm. ( b ) Image sequence showing a single granule undergoing exocytosis; 1 or 0.1 s between images, as indicated. ( c ) Quantification of experiments in a , b . Average fluorescence time course of all exocytosis events (Δ F ), aligned to the time of exocytosis and normalized to cell brightness ( F ); 68 granules in 8 cells. ( d ) Quantification of docking, visiting, exocytosis and failures in a , b . ( e ) NPY-cherry-expressing cells imaged in TIRF and Epi mode, and colour overlay as indicated. The TIRF image was acquired 50 ms after the Epi image. Scale bar, 2 μm. ( f ) Scatterplot of the TIRF versus Epi signals at granules (Δ F ). Each point represents a granule. ( g ) Histogram of the TIRF/Epi ratio for the data in f , scaled as height from the coverslip using a decay constant of 100 nm and assuming that the peak represents granules touching the plasma membrane. ( h ) Cells expressing NPY-cherry (TIRF, Epi) and syntaxin-EGFP (Syx) were imaged in TIRF and Epi mode and stimulated with K + . Examples of docking, exocytosis (exo) and visiting events are shown. The syntaxin signal was acquired 100 ms before the granule images. Scale bar, 1 μm. To emphasize changes in granule-associated fluorescence, the image sequences were linearly scaled for best contrast. ( i ) Quantification of the TIRF/Epi ratio for granules as in h . The TIRF Δ F signal was divided by the average Epi Δ F signal during 5 s before (exocytosis, failures) or after (docking, visiting) the event. Failures are time-matched granules that did not undergo exocytosis. Data from 20–49 granules in 5–11 cells. Full size image Some of the granules undergoing exocytosis may have been arrested slightly above the plasma membrane, for example by the actin cortex. Since TIRF-M is not an absolute measure of granule distance to the membrane, we modified the microscope to allow for rapid switching between Epi and TIRF mode ( Fig. 2e ). In Epi mode the granule brightness is little affected by variations in axial distance, and the TIRF/Epi fluorescence ( T/E ) ratio can therefore be used to normalize the TIRF signal and to calculate relative distances. Zero distance from the membrane is given by granules that undergo exocytosis. T and E values for granules were linearly related ( Fig. 2f ) and the T/E ratio demonstrates that fewer than 5% of visible granules were further than 50 nm from the plasma membrane ( Fig. 2g ). We again observed docking, visiting and exocytosis events in cells stimulated with K + and aligned the granule’s T/E ratio to these events ( Fig. 2h,i ). Granules undergoing exocytosis had T/E ratios very similar to docked granules that did not exocytose (failures), indicating that they were localized at the membrane. Visiting granules also reached T/E ratios similar to those observed before exocytosis, suggesting that these granules likewise reached the membrane. The s.d. of the signal at docked granules was 44 nm. It is therefore unlikely that more than a few of these granules were tethered by other means than through interaction with the plasma membrane. Indeed, destruction of the actin cortex did not affect the density of docked granules ( Supplementary Fig. 3 ). Syntaxin clusters form during docking We then investigated how syntaxin clusters develop during docking and visiting events. Surprisingly, none of 33 docking and 43 visiting events (14 cells) occurred at a pre-existing syntaxin cluster ( Fig. 3j , before). Instead, syntaxin clusters could be seen to form at the contact site just after arrival of stably docking granules ( Fig. 3b,j docking). We temporally aligned the syntaxin Δ F/S signal to the moment of granule contact with the docking site ( Fig. 3d , docking). The onset of syntaxin recruitment coincided with the moment of granule contact with the plasma membrane; before this time point the average was indistinguishable from zero. It then reached Δ F/S ≈0.1 within 5 s after docking, identical to the average for already docked granules ( Fig. 3i , ‘visible’) and indicating that most syntaxin is recruited during docking. Two-thirds of granules that stably docked acquired a visible cluster during the first 10 s at the plasma membrane ( Fig. 3j , dock), compared with ~80% of already docked granules ( Fig. 3j , visible). Since most of this occurred a few seconds after the granule reached the plasma membrane, it is likely that the granule initiates clustering of syntaxin at the docking site. In contrast, visitor granules failed to recruit syntaxin during their presence at the plasma membrane, even when they remained tethered for longer than the ~5 s required for syntaxin cluster formation ( Fig. 3b,d,i,j , visiting). This suggests that syntaxin clusters form as part of the docking process and that granule contact with the plasma membrane is required but not sufficient for this to occur. It is not clear why there was a slight tendency for exclusion of syntaxin from the visited sites, resulting in negative Δ F/S . 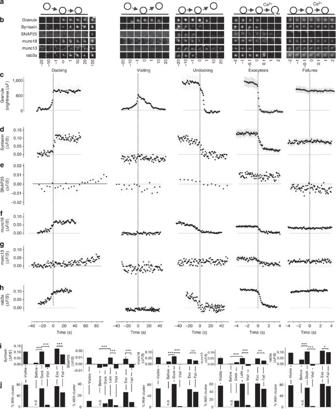Figure 3: Time course of protein binding during granule events. (a) Cartoons illustrating granule docking, visiting, undocking, exocytosis and failure events. (b) Example image sequences of granule marker and EGFP-labelled syntaxin-1, SNAP25, munc18, munc13 and rab3a during granule events as indicated; images are centred on the granule position in the docked/tethered state. Docking and visiting was recorded at 1 s−1and exocytosis at 10 s−1. Scale bar, 0.5 μm. To emphasize changes in granule-associated fluorescence, the image sequences were linearly scaled for best contrast. Note that since out-of-cell background is not shown, ΔF/Scannot be calculated from the displayed images. (c) Quantification of granule brightness; from the same cells as inb. Data were recorded at 1 s−1and are temporally aligned to granules events as indicated by vertical dotted lines. (d–h) Quantification of protein binding to the docking site (ΔF/S), temporally aligned to granule events as indicated. Scales apply to all graphs in the respective row or column. Positive ΔF/Svalues indicate specific binding of the protein to the docking site, negative values indicate exclusion. Note that for partially cytosolic proteins the volume of the granules leads to exclusion; for EGFP alone this amounts to ΔF/S=−0.006±0.001. ΔF/Sat random locations was −0.003±0.005 for syx, −0.031±0.005 for SNAP25, 0.002±0.006 for M18, 0.001±0.004 for M13. A total of 20–68 granules from 9–44 cells for each condition. SeeSupplementary Fig. 4A,Bfor individual examples. Data for SNAP25 are shown on a different ordinate scale and binned for clarity. SeeSupplementary Fig. 6for example images. For syntaxin, all points att≥0 s (except 1 s) were significantly higher than the pre-docking average at −10<t<−6 s, while no difference was detected for points att<0s (allP>0.5). (i) Bar graphs showing average ΔF/Svalues during the time intervals indicated. ‘Docked’ refers to granules that remained docked throughout the experiment. ‘Before’ refers to the 20 s interval before a docking event, ‘docking’ to the 20 s interval after the granule arrived and stayed >25 s, ‘Visiting’ refers to the 10 s interval after a granule arrived and stayed for 10–25 s. ‘Exocytosis’ and ‘Failures’ refers to 2-s interval before exocytosis. The latter are pairwise time-matched to exocytosis events. The time point >120 s was not assessed for syx, Munc18 and Rab3. SeeSupplementary Fig. 4Cfor additional analysis. (j) Observer-based quantification of cluster colocalization with the docking site for events as ind–hin average images of the intervals as ini. Figure 3: Time course of protein binding during granule events. ( a ) Cartoons illustrating granule docking, visiting, undocking, exocytosis and failure events. ( b ) Example image sequences of granule marker and EGFP-labelled syntaxin-1, SNAP25, munc18, munc13 and rab3a during granule events as indicated; images are centred on the granule position in the docked/tethered state. Docking and visiting was recorded at 1 s −1 and exocytosis at 10 s −1 . Scale bar, 0.5 μm. To emphasize changes in granule-associated fluorescence, the image sequences were linearly scaled for best contrast. Note that since out-of-cell background is not shown, Δ F/S cannot be calculated from the displayed images. ( c ) Quantification of granule brightness; from the same cells as in b . Data were recorded at 1 s −1 and are temporally aligned to granules events as indicated by vertical dotted lines. ( d – h ) Quantification of protein binding to the docking site (Δ F/S ), temporally aligned to granule events as indicated. Scales apply to all graphs in the respective row or column. Positive Δ F/S values indicate specific binding of the protein to the docking site, negative values indicate exclusion. Note that for partially cytosolic proteins the volume of the granules leads to exclusion; for EGFP alone this amounts to Δ F/S =−0.006±0.001. Δ F/S at random locations was −0.003±0.005 for syx, −0.031±0.005 for SNAP25, 0.002±0.006 for M18, 0.001±0.004 for M13. A total of 20–68 granules from 9–44 cells for each condition. See Supplementary Fig. 4A,B for individual examples. Data for SNAP25 are shown on a different ordinate scale and binned for clarity. See Supplementary Fig. 6 for example images. For syntaxin, all points at t ≥0 s (except 1 s) were significantly higher than the pre-docking average at −10< t <−6 s, while no difference was detected for points at t <0s (all P >0.5). ( i ) Bar graphs showing average Δ F/S values during the time intervals indicated. ‘Docked’ refers to granules that remained docked throughout the experiment. ‘Before’ refers to the 20 s interval before a docking event, ‘docking’ to the 20 s interval after the granule arrived and stayed >25 s, ‘Visiting’ refers to the 10 s interval after a granule arrived and stayed for 10–25 s. ‘Exocytosis’ and ‘Failures’ refers to 2-s interval before exocytosis. The latter are pairwise time-matched to exocytosis events. The time point >120 s was not assessed for syx, Munc18 and Rab3. See Supplementary Fig. 4C for additional analysis. ( j ) Observer-based quantification of cluster colocalization with the docking site for events as in d – h in average images of the intervals as in i . Full size image In the same movies, 21 additional granules undocked. These events can be distinguished from exocytosis because of their relatively slow time course and because no exocytosis was observed under these conditions. The frequency of undocking was similar to that of docking ( Supplementary Fig. 2B ). Undocking temporally coincided with loss of the syntaxin cluster ( Fig. 3a–d undocking); the average syntaxin signal fell from Δ F/S ≈0.1 to zero. Interestingly, the onset of the decay in the syntaxin signal appears to precede undocking, by on average 13±3 s ( Supplementary Fig. 4D , 21 events). In summary, the data suggest that syntaxin is recruited during the conversion of granules from a loosely tethered to the stably docked state, which in turn is required for exocytosis. Clustering of other proteins at the docking site We quantified several other exocytosis proteins at the docking site. SNAP25 has a relatively weak tendency to occupy clusters beneath docked granules [36] , resulting in Δ F/S ~0.01 ( Fig. 3i ) and clusters visible on 8% of granules ( Fig. 3j , visible). Before and just after arrival of the granule, EGFP-tagged SNAP25 was not detectable at the docking site ( Fig. 3i,j , before and dock); the site then slowly (1–2 min) accumulated the protein to similar amounts as found at already docked granules ( Fig. 3e,i,j late). Visitors did not attract SNAP25, and the protein was lost from the granule site during undocking ( Fig. 3e ). Munc18 is required for docking and binds syntaxin by clasping the auto-inhibited closed conformation [37] or by binding to a short N-terminal peptide. EGFP-tagged munc18 clustered at docked granules ( Fig. 3b,f and Supplementary Fig. 1B,D,F ), confirming recent super-resolution experiments [32] . Munc18 was initially absent from the docking site ( Fig. 3f,i before). After docking the munc18 signal increased and reached within seconds ΔF/S~0.05, identical to the average value for already docked granules ( Fig. 3i ). At the same time, clusters became detectable at ~80% of these granules. Like syntaxin, munc18 was not detected during visiting events ( Fig. 3f,i,j visiting), and was lost from the docking site during undocking ( Fig. 3f undocking). We noted that munc18 became already detectable during granule approach, likely because some granules arrive carrying munc18 with them ( Fig. 4a,b,e,g,h ). 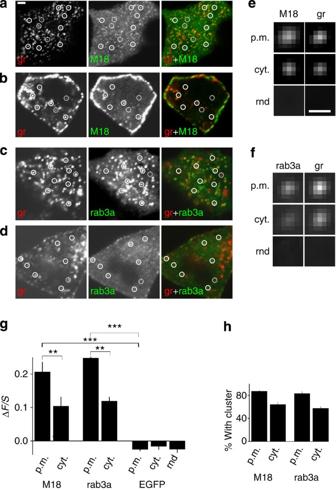Figure 4: Munc18 and rab3a colocalize with granules deeper in the cell. (a–d) Ins1 cells expressing NPY cherry (gr) and munc18-EGFP (M18,a,b) or EGFP-rab3a (rab3,c,d) were imaged by confocal microscopy.aandcwere recorded near the coverslip,banddwere recorded near the centre of the cell. Granules that colocalize with M18 or rab3a (circles), or not (dotted circles) are highlighted. Scale bar, 2 μm. (e) Spatially aligned average images for granule (gr) and munc18 (M18) and centred on either granules near the plasma membrane as ina(p.m.), granules away from the plasma membrane as inb(cyt) and random locations inb(rnd); >200 granules from >10 cells each, from six (M18) and three coverslips (rab3). Scaling to 8-bit for display was done with identical settings for all images, after first normalizing for the average background-subtracted annulus fluorescence (S). Scale bar, 0.5 μm. (f) As inebut for rab3a. (g) Quantification of binding to the granule site (ΔF/S) for munc18, rab3a and EGFP as control. (h) Observer-based quantification of cluster association with granules for rab3a and munc18. Figure 4: Munc18 and rab3a colocalize with granules deeper in the cell. ( a – d ) Ins1 cells expressing NPY cherry (gr) and munc18-EGFP (M18, a , b ) or EGFP-rab3a (rab3, c , d ) were imaged by confocal microscopy. a and c were recorded near the coverslip, b and d were recorded near the centre of the cell. Granules that colocalize with M18 or rab3a (circles), or not (dotted circles) are highlighted. Scale bar, 2 μm. ( e ) Spatially aligned average images for granule (gr) and munc18 (M18) and centred on either granules near the plasma membrane as in a (p.m.), granules away from the plasma membrane as in b (cyt) and random locations in b (rnd); >200 granules from >10 cells each, from six (M18) and three coverslips (rab3). Scaling to 8-bit for display was done with identical settings for all images, after first normalizing for the average background-subtracted annulus fluorescence ( S ). Scale bar, 0.5 μm. ( f ) As in e but for rab3a. ( g ) Quantification of binding to the granule site (ΔF/S) for munc18, rab3a and EGFP as control. ( h ) Observer-based quantification of cluster association with granules for rab3a and munc18. Full size image Munc13 is required for synaptic vesicle exocytosis [38] and binds directly to both syntaxin and munc18 (refs 39 , 40 ). About half of all visible granules colocalized with munc13-EGFP clusters ( Fig. 3j visible, and Supplementary Fig. 1C,D,F ), resulting in Δ F/S ~0.05 for already docked granules. No munc13 was detected before arrival of a granule ( Fig. 3i before). Unlike syntaxin, the munc13 signal then only slowly increased ( Fig. 3g ) and remained near zero up to 40 s after docking ( Fig. 3g docking). It then increased slowly and after 2 min reached the same Δ F/S and cluster association as found on already docked granules ( Fig. 3i,j late). Refilling of the RRP in mouse β-cells by priming takes ~60 s (ref. 41 ). The late recruitment of munc13 is therefore consistent with its role in granule priming rather than docking [42] , although the relationship may not be causal. Munc13 was not detected during visiting events ( Fig. 3g,i,j visiting). Rab3a is a granule-associated small GTPase that is known to bind munc18 and has been implicated in docking [22] , [23] . As expected, EGFP-labelled rab3a was found on granules, both near the plasma membrane and deeper within the cell ( Fig. 3h , visible, Fig. 4c,d,f–h ). Consequentially, the rab3a signal increased during the approach of the granule but did not increase further once the granule had reached the plasma membrane ( Fig. 3h–j , dock), and the rab3a signal disappeared during undocking ( Fig. 3h undocking). Visitor granules did not carry or recruit rab3a, perhaps suggesting that the protein is involved in the signalling required to convert tethered granules to the stably docked state ( Fig. 3h–j , visit). Protein accumulation during granule priming To test how recruitment of these proteins is related to granule priming and the RRP, we evoked exocytosis similar to Fig. 2a–c . Docked granules that underwent exocytosis ( Fig. 3c , exocytosis) could then be compared with those that did not ( Fig. 3c , failures). Exocytosis granules, reflecting the primed pool (RRP, see Supplementary Fig. 2B ), had almost twice as much associated syntaxin (Δ F/S ) and a higher fraction colocalized with syntaxin clusters than time-matched failures ( Fig. 3i,j ). This indicates that the amount of syntaxin in the cluster affects release probability. Granules that underwent exocytosis also accumulated more munc18, SNAP25 and munc13 in their associated clusters than the failures ( Fig. 3e–g,i,j ), while rab3a was similar for both groups ( Fig. 3h ). Most of the cluster proteins were rapidly lost (<1 s) from the docking site during exocytosis, with the exception of SNAP25 and a fraction of the syntaxin. Assuming 50–70 syntaxin molecules per cluster [29] , [30] , [31] , the latter corresponds to <20 syntaxin molecules remaining at the exocytosis site, which could reflect cis SNARE complexes formed during exocytosis. A soluble syntaxin Habc fragment disperses the docking site protein cluster Syntaxin clusters associate with granules via the N-terminal Habc domain, independent of the processes that lead to self-aggregation of syntaxin; a truncated syntaxin lacking this domain (SyxΔHabc) forms clusters that do not associate with granules ( Fig. 5a–c and refs 36 , 43 ). This provides an opportunity to test how docking is affected when syntaxin clusters cannot form at granules. A soluble Habc fragment (syntaxin 1A 1–159) was designed to compete with syntaxin for binding to the docking site. The fragment and granule marker were expressed from a bicistronic IRES vector, together with syntaxin-EGFP ( Fig. 5a–c ). As expected, the Habc fragment interfered with association of syntaxin-EGFP with granules, and Δ F/S was reduced to less than half compared with control. The Habc fragment did not affect expression or membrane targeting of syntaxin-EGFP, and off-granule clusters were still present ( Fig. 5a and Supplementary Fig. 5A,B ). Interestingly, the Habc fragment also prevented munc18 and munc13 from binding to the docking site ( Fig. 5a–c ), and munc18 bound to clusters of syntaxin, but not syntaxin-ΔHabc ( Supplementary Fig 6G–I ). 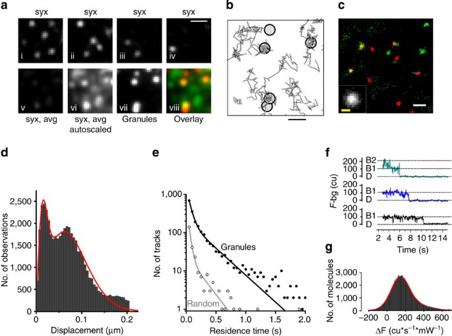Figure 6: Syntaxin clusters arise from short temporary binding of single molecules to the docking site. (a) Single-molecule imaging of Syx-EGFP at 50 Hz. (i–iv) Examples of the syntaxin channel (syx) showing single molecules at different time points in the same cell, (v) the movie average of the syntaxin channel, (vi) contrast-enhanced movie average, (vii) granule channel and (viii) overlay of vi and vii. Images are lowpass filtered (3 × 3) for display. Images i–v are linearly scaled with identical settings so that contrast is optimized in image i. Scale bar, 1 μm. (b) Trajectories of individual syntaxin molecules (dotted lines) and granule positions (large circles) for the same area as ina. Note that some tracks are temporally confined near granules. Only tracks >1 s length are included. Scale bar, 0.5 μm. (c) Super-resolution image of syntaxin-EGFP and granule positions. The inset shows the spatial average of 74 syntaxin clusters (5 cells); inset scale bar, 100 nm. The average full-width at half maximum (FWHM) of these clusters was 103±4 nm, by fitting 2D-Gaussian functions. Scale bar, 0.5 μm. (d) Histogram of single molecule distance travelled per frame (50 ms). The red line is a fitted diffusion equation withD1=0.002 andD2=0.039 μm2s−1as diffusion coefficients. The minor peak at 0.2 μm is due to misassignment during tracking. (e) Histogram of single molecule residence times within circles of 300 nm diameter and centred at either granule (black) or random positions (hollow symbols). The distributions are significantly different (Kolmogorov–Smirnov test,P=2 × 10−10). The lines are global double exponential fits to the data with shared time constants of 51 and 273 ms; the contribution of the longer time constant reflecting binding to the granule was 14% at granule locations and 1.4% at random locations. In all, 1,101 tracks (>1 s length) and 325 granules, in 6 cells. (f) Three examples of step-wise bleaching (same cell asFig. 4a; average fluorescence in a 3 pxl wide circle). In the green example more than one molecule was initially present, of which the last bleached at 6 s. (g) Histogram of single molecule intensities subtracted with the local background (ΔF). Overlayed is the sum of two Gaussians with peaks at ΔF=140 and 247 camera units (cu), indicating single molecule fluorescence of 140 cu for a 50 ms exposure at 20 mW illumination (140 cu × s−1× mW−1,Fig. 4f). 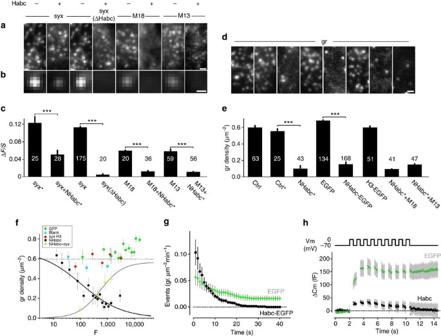This is consistent with the ability of munc13 and munc18 to bind to the Habc domain of syntaxin [40] and suggests that that both proteins are recruited into the cluster by binding to syntaxin. Figure 5: Syntaxin Habc fragment prevents granule-associated clusters and docking. (a) Representative images from cells expressing EGFP-labelled syntaxin (syx), truncated syntaxin (syx-ΔHabc), munc18 (M18) and munc13 (M13) in presence (+) or absence (−) of the Habc fragment. Conditions as indicated inc. All cells also expressed the granule marker (not shown). Scale bar, 1 μm. (b) Average images of the EGFP channel spatially aligned to granule locations, from images as ina. Ina,b, scaling to 8-bit for display was done with identical settings, after first normalizing for the average background-subtracted annulus fluorescence (S). Scale bar, 0.5 μm. (c) Quantification of binding to the docking site (ΔF/S) for proteins as in A. NHabc refers to co-expression of the N-terminal syntaxin fragment; asterisk indicates use of the bicistronic IRES vector. Fora–c: 20–175 cells from 3–5 coverslips each, as indicated. (d) Representative images showing granules (gr), for conditions as ine. Scale bar, 1 μm. (e) Quantification of granule density from images as ind. With granule marker only (ctrl), or together with Habc, EGFP or EGFP-tagged Habc, H3, M18 or M13 as indicated. A total of 25–168 cells from 3–5 coverslips each; asterisk indicates use of the bicistronic IRES vector. (f) Granule density as function of expression level of EGFP (green circles), pIRES control (blue triangles), H3-EGFP (red diamonds), NHabc-EGFP (black squares). Expression is measured as background-subtracted average EGFP fluorescence in the cell (F). Black line is a Hill equation fit to the Habc-EGFP data set; dotted line is the average for granule marker only. Yellow triangles show cells expressing NHabc, as function of Syx-EGFP expression; grey line is a Hill equation fit to this data set. Symbols represent averages of 10 cells each. (g) Scaled survival plot of granule residence times as inFig. 1b, in cells coexpressing granule marker with EGFP (green; 105 granules, 6 cells) or Habc-EGFP (black; 177 granules, 12 cells). (h) Whole-cell capacitance measurements of exocytosis for cells expressing Habc-EGFP (black dots) or EGFP (green dots); 7 cells each. Solid line shows the voltage-clamp protocol. Figure 5: Syntaxin Habc fragment prevents granule-associated clusters and docking. ( a ) Representative images from cells expressing EGFP-labelled syntaxin (syx), truncated syntaxin (syx-ΔHabc), munc18 (M18) and munc13 (M13) in presence (+) or absence (−) of the Habc fragment. Conditions as indicated in c . All cells also expressed the granule marker (not shown). Scale bar, 1 μm. ( b ) Average images of the EGFP channel spatially aligned to granule locations, from images as in a . In a , b , scaling to 8-bit for display was done with identical settings, after first normalizing for the average background-subtracted annulus fluorescence ( S ). Scale bar, 0.5 μm. ( c ) Quantification of binding to the docking site (Δ F/S ) for proteins as in A. NHabc refers to co-expression of the N-terminal syntaxin fragment; asterisk indicates use of the bicistronic IRES vector. For a – c : 20–175 cells from 3–5 coverslips each, as indicated. ( d ) Representative images showing granules (gr), for conditions as in e . Scale bar, 1 μm. ( e ) Quantification of granule density from images as in d . With granule marker only (ctrl), or together with Habc, EGFP or EGFP-tagged Habc, H3, M18 or M13 as indicated. A total of 25–168 cells from 3–5 coverslips each; asterisk indicates use of the bicistronic IRES vector. ( f ) Granule density as function of expression level of EGFP (green circles), pIRES control (blue triangles), H3-EGFP (red diamonds), NHabc-EGFP (black squares). Expression is measured as background-subtracted average EGFP fluorescence in the cell ( F ). Black line is a Hill equation fit to the Habc-EGFP data set; dotted line is the average for granule marker only. Yellow triangles show cells expressing NHabc, as function of Syx-EGFP expression; grey line is a Hill equation fit to this data set. Symbols represent averages of 10 cells each. ( g ) Scaled survival plot of granule residence times as in Fig. 1b , in cells coexpressing granule marker with EGFP (green; 105 granules, 6 cells) or Habc-EGFP (black; 177 granules, 12 cells). ( h ) Whole-cell capacitance measurements of exocytosis for cells expressing Habc-EGFP (black dots) or EGFP (green dots); 7 cells each. Solid line shows the voltage-clamp protocol. Full size image Successful docking, but not tethering, requires clustered syntaxin Consistent with the idea that syntaxin clusters are required for docking, co-expression of the Habc fragment reduced docked granules to one-sixth compared with control ( Fig. 5d,e ). Similarly, an EGFP-tagged Habc fragment (Habc-EGFP) associated with granules ( Supplementary Fig. 5D–F ) and reduced docked granule density to less than one-third of the EGFP control, while a fragment derived from the H3/SNARE domain of syntaxin (H3-EGFP) had little or no effect ( Fig. 5d,e ). Since the fluorescence of Habc-EGFP in each cell depends on its concentration, dose response relationships can be constructed. Figure 5f plots the granule density against the background-corrected cellular EGFP fluorescence. With EGFP, the granule density remained ~0.6 granules per μm 2 up to the highest fluorescence observed. In contrast, with Habc-EGFP the granule density decreased with increasing expression of the fragment to ~0.15 granules per μm 2 . Interestingly, the docking defect with Habc could be rescued dose-dependently by co-expression of syntaxin-EGFP ( Fig. 5f ), while co-expression of munc18-EGFP or munc13-EGFP did not rescue the docking defect caused by the Habc fragment ( Fig. 5d,e ), suggesting that high local concentrations of syntaxin, as in clusters, may be a critical requirement for stable docking. Visual inspection of movies of cells expressing the Habc fragment suggested that granules were still able to reach the PM, but they failed to transition into the docked state. Quantification of the docking site residence times showed that expression of Habc-EGFP essentially prevented stable docking events, while the total number of visiting events nearly doubled ( Fig. 5g ). Similar results were obtained with the unlabelled Habc fragment expressed from a bicistronic IRES vector ( Supplementary Fig. 5C ). Expression of EGFP as control resulted in normal residence times as with granule marker only ( cf. Fig. 1c ). Thus, when syntaxin clusters are prevented from forming near granules by the Habc fragment, stable docking is rare despite an increased frequency of docking attempts. This suggests that the initial tethering is still operational, but that the transition into the docked state fails. Expression of the Habc-EGFP also greatly reduced exocytosis, as measured by capacitance in cells stimulated with a train of voltage-clamp depolarizations ( Fig. 5h ). Both the initial capacitance increase, which reflects exocytosis of primed granules, and the summed increase during depolarizations 3–9, which reflects recruitment by docking and priming, were reduced to one-fourth of the EGFP control. This is consistent with the finding that deletion of the Habc domain results in fewer releasable vesicles in neurons [44] . Rapid exchange between clustered and free syntaxin molecules To understand the rapid aggregation of syntaxin during docking, we turned to single-molecule imaging of Syx-EGFP ( Fig. 6a ) [30] . Single syx-EFGP molecules exhibited step-wise bleaching ( Fig. 6f ) and unitary brightness ( Fig. 6a i–iv and f,g) and were highly mobile within the PM ( Fig. 6b,d ). Interestingly, when the recorded movies were time-averaged ( Fig. 6a v,vi), the staining pattern was similar to that seen at higher expression levels, including the appearance of punctate structures that partially colocalize with granules. The data allowed us to construct single-molecule localization microscopy (SMLM) images of syntaxin-EGFP ( Fig. 6c ), which showed clustered syntaxin-EGFP with an average width (FHWM) of 103±4 nm ( n =74). This is slightly larger than previous estimates of syntaxin cluster size (60–90 nm; refs 28 , 43 , 45 , 46 ), possibly due to the use of live rather than fixed cells or higher precision of the earlier measurements. Visually, two types of syntaxin behaviour were apparent: one of apparently random diffusion and another where molecules were temporarily confined to a small area, often beneath a granule ( Fig. 6b ). Analysis of the trajectories [47] revealed two dominant diffusion modes with diffusion coefficients of D 1 =0.002 and D 2 =0.039 μm 2 s −1 ( Fig. 6d ), which is similar to previous estimates in PC12 cells [30] . Residence times at the granule have not been estimated previously. We compared the single-molecule residence time at granules with that at random locations; in both cases the histogram could be fit with a double-exponential function, as would be expected for a mixture of bound and freely moving molecules ( Fig. 6e ). The longer of the two fitted time constants (273 ms) likely results from molecules that temporary bind at the analysed location. The fraction of these spatially confined molecules was 10-fold larger beneath granules than at random locations in the same cells ( Fig. 6e ). Thus, cluster-bound syntaxin molecules rapidly exchange with free molecules in the surrounding plasma membrane and short-term binding to the docking site explains the appearance of clusters. The average fluorescence of a single molecule was 140 camera units (cu) for a 50 ms exposure at 20 mW illumination (140 cu × s −1 × mW −1 , Fig. 6g ), compared with 4,090±390 cu × s −1 × mW −1 for the average syntaxin cluster in Fig. 3d ( n =31). This indicates that on average the clusters contained ~29 syntaxin-EGFP molecules. The average Δ F values in the data for Fig. 3f suggests 75±13 ( n =221) munc18-EGFP molecules per cluster. Figure 6: Syntaxin clusters arise from short temporary binding of single molecules to the docking site. ( a ) Single-molecule imaging of Syx-EGFP at 50 Hz. (i–iv) Examples of the syntaxin channel (syx) showing single molecules at different time points in the same cell, (v) the movie average of the syntaxin channel, (vi) contrast-enhanced movie average, (vii) granule channel and (viii) overlay of vi and vii. Images are lowpass filtered (3 × 3) for display. Images i–v are linearly scaled with identical settings so that contrast is optimized in image i. Scale bar, 1 μm. ( b ) Trajectories of individual syntaxin molecules (dotted lines) and granule positions (large circles) for the same area as in a . Note that some tracks are temporally confined near granules. Only tracks >1 s length are included. Scale bar, 0.5 μm. ( c ) Super-resolution image of syntaxin-EGFP and granule positions. The inset shows the spatial average of 74 syntaxin clusters (5 cells); inset scale bar, 100 nm. The average full-width at half maximum (FWHM) of these clusters was 103±4 nm, by fitting 2D-Gaussian functions. Scale bar, 0.5 μm. ( d ) Histogram of single molecule distance travelled per frame (50 ms). The red line is a fitted diffusion equation with D 1 =0.002 and D 2 =0.039 μm 2 s −1 as diffusion coefficients. The minor peak at 0.2 μm is due to misassignment during tracking. ( e ) Histogram of single molecule residence times within circles of 300 nm diameter and centred at either granule (black) or random positions (hollow symbols). The distributions are significantly different (Kolmogorov–Smirnov test, P =2 × 10 −10 ). The lines are global double exponential fits to the data with shared time constants of 51 and 273 ms; the contribution of the longer time constant reflecting binding to the granule was 14% at granule locations and 1.4% at random locations. In all, 1,101 tracks (>1 s length) and 325 granules, in 6 cells. ( f ) Three examples of step-wise bleaching (same cell as Fig. 4a ; average fluorescence in a 3 pxl wide circle). In the green example more than one molecule was initially present, of which the last bleached at 6 s. ( g ) Histogram of single molecule intensities subtracted with the local background (Δ F ). Overlayed is the sum of two Gaussians with peaks at Δ F =140 and 247 camera units (cu), indicating single molecule fluorescence of 140 cu for a 50 ms exposure at 20 mW illumination (140 cu × s −1 × mW −1 , Fig. 4f ). Full size image Our results confirm that syntaxin is essential for secretory granule docking. Importantly, the presence of syntaxin in the plasma membrane is not sufficient; it must also cluster at the docking site. We now show that syntaxin clusters form during successful docking events, and act as platform where the secretory machinery assembles. Contact of the granule with the plasma membrane induces within seconds the de novo formation of a syntaxin cluster, which in turn stabilizes the docked state. We provide strong evidence that acute clustering of syntaxin is required for docking. First, docking does not occur when clustering is prevented with the Habc fragment. Second, visiting granules fail to recruit syntaxin. Third, conversion into the docked state has a similar rate constant as syntaxin clustering. The data are consistent with a model ( Fig. 7 ) where factors on the granule organize the plasma membrane at the nascent docking site. This leads initially to clustering of syntaxin and munc18 from a pool of freely diffusing molecules. Munc18 is recruited at the same time. It is likely that munc18 recruitment depends on syntaxin [48] , because it is prevented with the soluble Habc fragment, and munc18 mutants deficient in syntaxin binding do not localize to the plasma membrane or support docking [18] , [48] . Additional proteins required for building the exocytosis machinery, such as munc13, SNAP25 and Ca 2+ channels, are then sequentially recruited to this site. 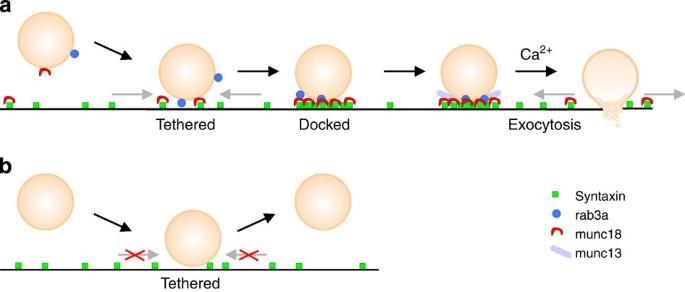Figure 7: Model of secretory granule docking. (a) Successful docking: The granule approaches the plasma membrane where it induces clustering of free syntaxin and munc18 molecules. Clustered syntaxin then stabilizes the docked state. Later, the site matures by recruiting additional proteins, allowing exocytosis. (b) Transition to the docked state does not occur when syntaxin/munc18 cluster formation fails, for example in presence of the Habc fragment. Figure 7: Model of secretory granule docking. ( a ) Successful docking: The granule approaches the plasma membrane where it induces clustering of free syntaxin and munc18 molecules. Clustered syntaxin then stabilizes the docked state. Later, the site matures by recruiting additional proteins, allowing exocytosis. ( b ) Transition to the docked state does not occur when syntaxin/munc18 cluster formation fails, for example in presence of the Habc fragment. Full size image Only one-third of the docking attempts are successful, but temporary tethering occurs even during failed attempts (visitors). Weak molecular interactions must therefore exist between granule and plasma membrane that do not require the syntaxin cluster. Indeed, synaptic vesicles are linked to the active zone membrane by short filaments or tethers of <40 nm (ref. 49 ). Recruitment of free syntaxin molecules can then rapidly convert the tethered granule into the stably docked state. The fact that this conversion often fails may reflect a stochastic effect where breaking the tether and undocking competes with recruitment of syntaxin and stabilization of docking; if syntaxin is late, the probability for undocking increases. Alternatively, granules may carry molecular cues that initiate syntaxin recruitment and confer weak interactions between granule and plasma membrane during the tethering phase [10] . Good candidates for this are the small GTPases Rab3 and Rab27, which are located on the granule. About half of the cytosolic granules carry rab3 ( Fig. 4 ), and only rab3-positive granules succeed to dock stably. Rab3 in turn binds munc18 (refs 19 , 43 , 45 ), which could provide a mechanism that recruits munc18 to the granule membrane [50] , in addition to its localization at the plasma membrane that depends on syntaxin [48] . Supporting this idea [50] , about half the granules deep in the cytosol are decorated with munc18 ( Fig. 4 ). Bound to the incoming granule, munc18 would be well positioned to initiate clustering of syntaxin in the plasma membrane, perhaps by directing syntaxins’ inherent tendency to self-aggregate [29] to the granule site. Together with syntaxin, additional munc18 is recruited during docking, because the munc18 signal continued to increase after arrival of the granule, and because undocked granules carry only half as much munc18 as those docked at the plasma membrane. Surprisingly, we do not observe docking at pre-existing syntaxin clusters. The clusters form only after arrival of the vesicle, which is difficult to reconcile with the notion that they act as molecular beacons [26] or docking receptor for the incoming granule. The latter has been proposed since PIP2 and PIP3 concentrate in syntaxin clusters [33] , [34] and affect clustering of syntaxin [26] , and since liposomes bind to syntaxin/PIP2 clusters in artificial bilayers [26] . However, acute clustering of PIP2 or PIP3 is not yet demonstrated in live cells and only 5–10% colocalization is reported between PIP2 and syntaxin decorated granules [33] , [34] . One possibility is therefore that clustering of these lipids is secondary to the self-aggregation of syntaxin. Alternatively, it can be speculated that either local activation of a lipid kinase by the granule or contact of the granule protein synaptotagmin with the plasma membrane [25] , [26] , [34] concentrates PIP2/PIP3 at the docking site. The latter would be consistent with the reported requirement for synaptotagmin during docking [17] , although direct binding between syntaxin and synaptotagmin cannot be important since synaptotagmin does not bind the Habc domain [51] . Mechanistically, formation of clusters requires that the protein is available in the surround, and indeed we find a lower density of the syntaxin in the vicinity of the granule. Depending on the true cluster size, the measured concentration of syntaxin in clusters is ~8–20-fold higher than in the vicinity (see Methods). PC12 cells contain ~75 molecules syntaxin per 50 nm cluster and an average syntaxin density of 500–1,800 μm −2 (refs 29 , 30 ). The latter corresponds to 1–3.6 syntaxin molecules randomly positioned in an area the size of the cluster, and ~20-fold concentration within the cluster during docking. Single-molecule imaging suggests that short-term binding events at the docking site are the underlying cause for this concentration. The conformation of syntaxin and SNAP25 in the clusters is not known. The proteins form a binary complex that is likely present in the clusters [24] and acts as acceptor for vesicle-bound synaptobrevin [19] , [35] . Formation of this trimeric core complex could therefore play a role in syntaxin clustering and docking by bridging granule and plasma membrane. However, this is unlikely because clustering is not affected by cleavage of synaptobrevin with tetanus toxin [36] , and proceeds independently of the amount of SNAP25 in the cluster ( Fig. 3 ). Further, inclusion of the H3 domain does not affect docking, although it interferes with core complex formation and blocks exocytosis [52] . Alternatively, the H3 fragment could interact directly with the central cavity of Munc18, where it competes with the SNARE four-helix bundle [53] . The resulting syntaxin (Habc)+H3 bundle would conceivably still recruit Munc18 into the complex. It is not clear why the bulk of munc13 and SNAP25 is recruited much later than syntaxin. The timing is consistent with a role in priming rather than docking, and both proteins are enriched at release-ready granules. Munc13 binding to the plasma membrane depends on PIP2 and Ca 2+ (ref. 54 ) and we noticed rapid depolarization-induced recruitment of munc13 to the membrane, although specific recruitment to the docking site might still depend on accumulation of PIP2 within the clusters [33] , [34] . Such a mechanism would provide a convenient explanation for the dependence of priming on munc13, PIP2 and Ca 2+ . While basal munc13 levels in the plasma membrane are sufficient for slow recruitment, increased availability in the plasma membrane (Ca 2+ ) and affinity to the release site (PIP2) would accelerate munc13 accumulation at the release site. Another possibility is the involvement of the rab3 effector Rab-interacting-molecule RIM1 (ref. 51 ), which in turn binds munc13 (ref. 55 ) and SNAP25 (ref. 56 ) and could direct these proteins to the release site. We observed striking differences in the amount of SNAP25 or munc13 between clusters, likely as a consequence of slow recruitment. This may in part explain why the interaction between syntaxin and SNAP25 (measured as FRET) varies from cluster to cluster [45] . Glucose-induced insulin secretion is biphasic, with a rapid 1st phase followed by a slower sustained 2nd phase. These biphasic release kinetics are physiologically relevant for insulin action and are thought to result from a limited pool of releasable granules that is slowly replenished by granule priming. Second-phase secretion is not observed in the absence of glucose, which reflects the ATP-dependence of insulin granule priming [8] . The subcellular location where priming takes place is debated. Stimulated secretion reduces docked insulin granules [5] and repeated stimulation by patch clamp depolarizations releases only a fraction of the docked granules [2] , [4] . We confirm this here by showing that release of all primed granules leaves at least half of the docked granules in place. In chromaffin cells, a few granules (15%) are in a dead-end docked state and remain resistant to repeated stimulation [4] , and we would not be surprised to find this also in Ins1 cells. In contrast, immediate exocytosis of newly arriving insulin granules (crash fusion) has been observed by some authors [12] , [57] , [58] , but not others [2] , [4] , [6] , particularly during 2nd phase secretion. The finding suggests that some granules may be able to prime before docking. Crash fusion depends on syntaxin3 rather than on syntaxin1 (ref. 57 ) and could therefore represent an alternative mode of insulin granule exocytosis [12] that may be relevant during mild or sustained stimulation. Our stimulation protocol combines K + - and glucose stimulation, and leaves 2nd phase secretion intact [59] . Under these conditions, we do not observe exocytosis of visitor granules or crash fusion, and granules are docked for extended periods (minutes) before becoming release-competent. Although crash fusion has been reported in Ins1 cells [57] , it is possible that our failure to detect it here may be cell line- or protocol-specific. While Ins1 cells exhibit robust biphasic release kinetics [60] akin to isolated rodent islets and have similar docked granule density, overall they contain fewer granules than primary β-cells. This may result in fewer visiting events and decrease the chance of visitor or crash fusion exocytosis. Alternatively, strong stimulation by the combination of glucose or ATP with forced depolarization may favour release of pre-docked granules at the expense of crash fusion. However, the biphasic nature of insulin secretion is well explained by the slower rate of priming relative to fusion, and docking is not rate limiting for the first few hours of insulin stimulation [5] , [61] . Docking defects would therefore be expected to result in fewer granules available for both 1st and 2nd phase secretion. This is relevant since SNARE proteins are reduced in diabetic islets [62] , which should directly affect docking and could account for secretory defects in patients with type-2 diabetes. The docking step is therefore an attractive target for drug development that does not shortcut the physiological triggering mechanisms for insulin granule exocytosis. Cells Ins1 cells are a well-established rat insulinoma model of dense core granule exocytosis and insulin secretion; we used clone 832/13 (ref. 63 ) (kind gift from H. Mulder, Malmö). Cells were maintained in RPMI 1640 (Invitrogen) containing 10 mM glucose and supplemented with 10% fetal bovine serum, streptomycin (100 μg ml −1 ), penicillin (100 μg ml −1 ), Na-pyruvate (1 mM) and 2-mercaptoethanol (50 μM). The cells were plated on polylysine-coated coverslips, transfected using Lipofectamine 2000 (Invitrogen) and imaged 24–42 h later. Plasmids The constructs used were rat Munc13-EGFP (ref. 64 ); rat syntaxin-EGFP (ref. 36 ), rat EGFP-Rab3a (ref. 65 ), rat SNAP25-EGFP (ref. 36 ), rat syntaxin (180–288)-EGFP here referred to as ΔNT (ref. 36 ), pEGFP-C1 (Clontech) and human NPY-EGFP (ref. 36 ). The latter labels >80% of insulin granules 36 h after transfection, as determined by immunostaining for insulin. Mouse Munc18-EGFP was obtained by PCR amplification from a mouse brain cDNA library; the amplified mouse Munc18-1 gene was cloned into pEGFP-N1 using EcoR1 and Apa1. The resulting linker sequence is: KTDEEIS S RARDPPVAT M . S and M (in bold) are the end of the Munc18-1 gene and start of EGFP, respectively. X-IRES NPY-mCherry, where the first slot of the bicistronic vector is empty, was obtained by inserting PCR-amplified NPY-mCherry vector into the second multiple cloning site (MCS) of the pIRES vector (Clontech). Rat Syx (1–156), referred to as Syx NHabc, was synthesized (Genewiz, USA) and inserted in to the first MCS of X-IRES-NPY-mCherry to generate NHabc-IRES-NPY-mCherry. NHabc-EGFP was generated by cloning the same fragment into pEGFP, using Age1 and Not1; the resulting linker is TGRN M . Rat Syx-H3-EGFP (amino acids 191–255) was obtained by replacing mRFP with EGFP in Syx-H3-mRFP (ref. 66 ) using Age1 and Not1 sites. All constructs were verified by sequencing (MWG Operon, Germany). Syntaxin 1a-EGFP supports exocytosis and docking, forms clusters that overlap with endogenous syntaxin-1 clusters [29] , [31] , and enters into SNARE complexes in vitro [66] and in cells [24] . Estimates of the number of syntaxin molecules per cluster using syntaxin-EGFP are strikingly similar to those derived using antibodies [29] , [30] , and C-terminally EGFP-tagged syntaxins are known to sort correctly [67] . Syntaxin was C-terminally labelled, resulting in EGFP being on the outside of the plasma membrane. Note that an N-terminal fusion where EGFP is adjacent to the Habc domain has been reported to be excluded from the docking site [68] . Munc18-EGFP rescues hormone secretion after siRNA-mediated knockdown of Munc18-1 and Munc18-2 in PC12 cells [18] . Munc13-EGFP rescues defective priming and exocytosis in a mouse model lacking Munc13 (ref. 64 ). Solutions Cells were imaged in a solution containing (in mM) 138 NaCl, 5.6 KCl, 1.2 MgCl 2 , 2.6 CaCl 2 , 3 D-glucose and 5 HEPES (pH 7.4 with NaOH). Exocytosis was not observed under these conditions ( Supplementary Fig. 2B ). For exocytosis experiments the buffer instead contained 10 mM glucose and was supplemented with 2 mM forskolin and 200 μM diazoxide, a K + -ATP channel opener that prevents glucose-dependent depolarization. Exocytosis was then evoked by computer-timed local application of high K + (75 mM KCl equimolarly replacing NaCl) through a pressurized glass electrode similar to those used for patch clamp experiments. All experiments were carried out with constant buffer perifusion at 32 °C, except in Fig. 6 and Supplementary Fig. 1A–D . Microscopy Cells were imaged using custom-built lens-type total internal reflection (TIRF) microscopes based on an Axiovert 135 microscope with a × 100/1.45 objective (Carl Zeiss). Excitation was from two DPSS lasers at 561 nm and 473 nm (Cobolt, Stockholm, Sweden), controlled with an acousto-optical tunable filter (AOTF, AA-Opto, France) and using dicroic Di01-R488/561 (Semrock). The decay constant of the TIRF field was 100–110 nm, calculated using exit angle of the laser from the objective (through a glass hemisphere) and assuming an index of 1.37 in the cytosol. Cells were identified using only 561 nm light, to avoid bleaching of the EGFP signal. The emission light was separated onto the two halves of a 16-bit EMCCD camera (Roper Cascade 512B, gain setting at 3,800 arbitrary units throughout) using an image splitter (Optical Insights) with a cutoff at 565 nm (565dcxr, Chroma) and emission filters (FF01-523/610, Semrock; and ET525/50m and 600EFLP, both from Chroma). Scaling was 160 nm per pixel (pxl), except in Fig. 5a–e (100 nm). For display, images were linearly scaled to 8-bit. In Figs 1b,h,i and 3 , and Supplementary Fig. 2A–D exposure was 1 s at 473 nm (0.1 mW) and 561 nm (0.02 mW) simultaneously, resulting in 12±3% apparent GFP bleaching over 3 min. In Figs 1a,c and 3 exposure time was 100 ms in stream mode and simultaneously illuminated with 473 nm (1 mW) and 561 nm (0.1 mW). In Fig. 1f,g (time-lapse), image pairs of the two colour channels were acquired sequentially, first with 473 nm excitation (0.5 mW) for 1 s immediately followed by 561 nm (2 mW) for 100 ms. In Figs 3i,j (visible) and 5a–f the cells were exposed to 473 nm (1 mW) at 50 × 20 ms exposure and averaged, immediately followed by exposure to 561 nm (1 mW) for 100 ms. Figure 5g and Supplementary Fig. 5C were acquired by exciting with 561 nm (0.02 mW) at 1 s exposure followed by an image with 473 nm (0.1 mW) to verify expression of the EGFP-tagged fragment. Figures 2e–i was acquired on a custom-built AxioVert D1 microscope with a × 100/1.45 objective (Carl Zeiss) that allowed rapid switching between lens-type TIRF and Epi illumination. TIRF illumination was from two AOTF-controlled DPSS lasers at 561 nm and 491 nm (Cobolt, Stockholm, Sweden). Epi illumination was from a diode (MCWHL5, Thorlabs) coupled into the illumination path using a 50/50 beam splitter. Exposures were sequentially 50 ms Epi (561 nm), 50 ms TIRF (561 nm), 100 ms TIRF (491 nm). Filters sets were Chroma (Bellows Falls, VT, USA) parts zet405/488/561/640x, zet405/488/651/640m, ET525/50m, ET600/50m, zt405/488/561/640rpc. Confocal microscopy in Fig. 4 was done with a Zeiss LSM780 using a × 63/1.40 objective (Zeiss) with sequential scanning of the red (excitation 561 nm, emission 578–696 nm) and green channel (excitation 488 nm, emission 493–574 nm). Pinhole size was 0.61 μm, corresponding to 1 Airy unit. Images were acquired in 16-bit at gain settings 750 for both channels and 0.11 μm per pxl. The alignment of the red and green images was recorded once every experimental session using 100 nm beads (Molecular Probes, Eugene, OR, USA) immobilized on the coverslip surface and fluorescing in both channels. An algorithm programmed in Matlab was then used to shift, rotate and shrink the red image [69] ; residual misalignment in the bead images was 0.25+/−0.02 pxl (1,492 beads in 6 image pairs). Image analysis Colocalization of EGFP-labelled proteins with granules was quantified as described previously [36] . Granules that were well separated from other granules and the edge of the cell were identified (7–36 per cell), and their locations transferred to the green channel. An algorithm implemented as MetaMorph journal then read the average pixel fluorescence in (1) a central circle ( c ) of 3 pxl (0.5 μm) diameter, (2) a surrounding annulus ( a ) with an outer diameter of 5 pxl (0.8 μm) and (3) a background area not including any cell (bg) (see Supplementary Fig. 1H for illustration). Since the docking site is far smaller than the resolution of the microscope, the circle will contain all of the fluorescence originating from it. It also contains fluorescence from molecules not bound to the docking site, which is estimated using a . To obtain the specific on-granule fluorescence Δ F , the annulus value ( a ) was therefore subtracted from that of the circle ( c ) (Δ F=c−a ). To obtain off-granule fluorescence, the annulus value was background-corrected ( S=a− bg). S represents the local unbound concentration of the labelled protein, and averaged for each cell, S is linearly related to its expression level. The relationship of Δ F versus S follows a one-site binding equation that reaches saturation at higher expression levels [30] . For relatively small S , the ratio Δ F/S is a convenient measure of protein binding to the docking site, which is independent of the expression level. Positive Δ F/S values indicate binding to the docking site, negative values indicate exclusion. Note that the latter can occur for proteins with cytosolic expression due to exclusion by the granule volume. For untargeted EGFP we find Δ F/S =−0.06 and visible exclusion from the granule ( Supplementary Fig. 5D ). Note that Δ F is given as per-pixel average for the entire 0.5 μm −2 circle, and Δ F/S values are seemingly small (0.1 for syntaxin) because the on-granule fluorescence originates from a small protein cluster (measured diameter 50–100 nm, area 0.002–0.008 μm 2 ). This fluorescence is detected in the circle c (diameter 0.48 μm, 5 pxl with total area 0.128 μm 2 ) as average pixel value. Assuming a cluster size of 100 nm, a value of Δ F/S =0.1 corresponds to at least 0.1 × 5 pxl × 0.128 μm 2 /0.008 μm 2 =8-fold enrichment over background. Assuming a cluster size of 50 nm, Δ F/S =0.1 corresponds to 20-fold enrichment in the cluster. For single images, Δ F/S values were averaged for each cell; for movies Δ F/S was calculated for every frame, and only cells with F >200 pxl were included in the analysis. As control, randomly selected regions in the cells were treated identically to granule regions. Cluster colocalization was also estimated by an observer, as follows. A journal in MetaMorph presented an observer (unaware of the image context) with square cutouts of the green channel (11 μm 2 ) that were centred on the position of each previously identified granule. The user then made a yes/no choice based on whether the centre of the nearest perceived cluster was within one pixel of the centre of the square, guided by an overlaid circle. When this approach was applied to movies, 20 frames before or after a granule event were averaged. Granule fluorescence was measured as Δ F for the granule channel. In Fig. 2c , the Δ F values were normalized using F =cell−bg, where cell is the average fluorescence in the cells’ footprint. In Fig. 2h,i the Tirf/Epi ratio was determined by dividing the Δ F value in TIRF mode with that obtained in Epi mode averaged for t =0–5 s after arrival (docking, visiting) or −5 to 0 s before (exocytosis, failures). Candidate docking or undocking events were found manually as granules that approached the TIRF field with an axial component and become laterally confined for at least two frames (see example Supplementary Fig. 7G ). In Fig. 1d,e granules were individually tracked by Gaussian fitting using ImageJ SpeckleTrackerJ [46] . We define docking as granules that remain confined least 25 s; visitors were those granules that remained for <25 s after appearing at the plasma membrane. Docked granules in Fig. 3 were all granules visible in the TIRF field. Undocking is defined as slow movement of a previously docked granule away from its docking site. Exocytosis events were detected manually based on sudden disappearance of the granule fluorescence, which is different from the very slow disappearance seen during undocking ( Supplementary Fig. 7A–F ). The moment of exocytosis is defined as the first significant change (2 s.d.) from the pre-exocytosis baseline. Failures are docked granules in the same experiments that did not undergo exocytosis during stimulation; they were randomly paired with exocytosis events and the same time interval was analysed for both. In Fig. 2c the average background outside the cell area (bg) was subtracted for every frame. Granule density was calculated using a script that used the built-in ‘find maxima’ function in ImageJ ( http://rsbweb.nih.gov/ij ) for spot detection. Single-molecule imaging Syntaxin-EGFP was expressed from a truncated CMV promoter (ΔCMV) together with NPY-mCherry, as previously reported [30] . Single molecules were TIRF-imaged at 20 s −1 in live Ins1 cells. Pixel size was 100 nm ( Fig. 6a–f ) or 160 nm ( Fig. 6g ). Background outside the cell area was subtracted for every frame, and molecule trajectories were then analysed using ImageJ plug-in Particle tracker [47] or QuickPALM [70] . Figure 6c was reconstructed from single molecule locations (green) and granule positions (red) using a bin size of 25 nm. Spots representing syntaxin clusters were then selected manually and fit with a 2D-Gaussian function to obtain full-width at half maximum. In Fig. 6d , diffusion coefficients were obtained by fitting the displacement histogram with the function where r is the displacement, t the acquisition time frame (50 ms), and D 1 and D 2 the diffusion coefficients. In Fig. 6e , residence times were calculated in Excel (Microsoft) as the time a molecule remained within a circle of 300 nm diameter that was centred on granules or random locations; the resultant histograms were fit with a double-exponential function with shared parameters for the time constants. Data for Fig. 6g were obtained with the same microscope as Fig. 3 , with identical camera gain setting. Single molecules were automatically identified in MetaMorph using ‘Find spots’ and their intensities calculated as Δ F , the average fluorescence in a circle of 3 pxl (0.5 μm) diameter subtracted with the average fluorescence in a surrounding annulus of 5 pxl (0.8 μm). Capacitance measurements Single-cell measurements of exocytosis were performed by patch clamp in the whole-cell configuration as described previously [2] , using an EPC-9 amplifier and Pulse software (HEKA Elektronik, Lambrecht, Germany). Cells were selected based on their green fluorescence. The intracellular solution consisted of (in mM) 125 Cs-glutamate, 10 NaCl, 1 MgCl 2 , 3 ATP-Mg, 0.1 cAMP, 0.05 EGTA and 10 HEPES (pH 7.15). The extracellular solution (EC) was (in mM) 138 NaCl, 5.6 KCl, 1.2 MgCl 2 , 2.6 CaCl 2 , 10 D-glucose, 0.2 diazoxide, 5 mM HEPES (pH 7.40), 2 μM forskolin and held at ~32 °C. Capacitance was measured using 1,000 Hz, 20 mV sine waves around −70 mV and offline calculation in Pulse. Exocytosis was evoked using a train of 9 × 500 ms depolarizations to 0 mV at 1 s −1 . Statistics Data are presented as mean±s.e.m. unless otherwise stated. Statistical significance was assessed using Students t -test for two-tailed, paired or unpaired samples, as appropriate. Significant difference is indicated by asterisks (* P <0.05, ** P <0.01, *** P <0.001). Nonlinear fitting was done using the Levenberg–Marquardt method in Origin (OriginLab, USA) or Matlab ( Fig. 6c ). How to cite this article: Gandasi, N. R. et al. Contact-induced clustering of syntaxin and munc18 docks secretory granules at the exocytosis site. Nat. Commun. 5:3914 doi: 10.1038/ncomms4914 (2014).